DNA replication timing and selection shape the landscape of nucleotide variation in cancer genomes Cancer cells evolve from normal cells by somatic mutations and natural selection. Comparing the evolution of cancer cells and that of organisms can elucidate the genetic basis of cancer. Here we analyse somatic mutations in >400 cancer genomes. We find that the frequency of somatic single-nucleotide variations increases with replication time during the S phase much more drastically than germ-line single-nucleotide variations and somatic large-scale structural alterations, including amplifications and deletions. The ratio of nonsynonymous to synonymous single-nucleotide variations is higher for cancer cells than for germ-line cells, suggesting weaker purifying selection against somatic mutations. Among genes with recurrent mutations only cancer driver genes show evidence of strong positive selection, and late-replicating regions are depleted of cancer driver genes, although enriched for recurrently mutated genes. These observations show that replication timing has a prominent role in shaping the single-nucleotide variation landscape of cancer cells. Cancer is a disease caused by somatic mutations in normal cells, including single-nucleotide variants (SNVs), small insertions, small deletions, amplifications and deletions of large genomic regions, and chromosomal translocations. Using next-generation DNA sequencing technologies, somatic mutations have been mapped for hundreds of cancer genomes [1] , [2] , [3] , [4] , [5] , [6] , [7] , [8] , [9] , [10] , with thousands more under way [11] . How such alterations influence the tumorigenesis is not completely understood. Tumorigenesis can be regarded as an evolutionary process, driven by somatic mutations and clonal selection [12] . The evolutionary framework has improved our understanding of the genetic basis of cancer [13] , [14] , [15] . Although the somatic evolution of cancer cells is reminiscent of the evolution of organisms, the two differ in many ways, such as timescale, effective population size, mutation rate, and outcome of the evolution [15] , [16] . Understanding differences between the two can improve our understanding of the genetic basis of cancer. In studying evolutionary dynamics, it is important to distinguish the process of mutations from that of selection. For large-scale genetic alterations, it is difficult to delineate the mutational process from influences of selection because a large-scale event often alter both functional and neutral regions; it is possible only by complex, indirect computational methods [17] , [18] . On the other hand, for small-scale mutations, it is straightforward to delineate the two; the underlying mutation rate can be directly inferred from the observed mutation frequency in functionally neutral, or nearly neutral, regions. Of small-scale mutations, single-nucleotide variation is one of the most abundant, functionally important source of evolution [1] , [2] , [3] , [4] , [5] , [6] , [7] , [8] , [9] , [10] , [13] , [19] , [20] . A recent study [21] examined spectrums of small-scale mutations in cancer genomes. They concluded that somatic mutations depend on individual genomic features, such as guanine-cytosine (GC) content and replication timing, in a weak manner. There are several aspects that require further investigations. First, they examined only three cancer genomes, so the breadth of the conclusion was limited. Second, they derived the conclusion that genomic features are poor predictors of the mutation rate based on a low R 2 of the linear regression fit. Importantly, they pooled the mutation frequencies from genic and non-genic regions, not distinguishing the influence of the mutational processes from that of selection. Here we characterize the mutational and selectional dynamics of cancer cell evolution from maps of SNVs in human cancer genomes. We found that somatic SNV frequency strongly increased with replication time during the S phase, suggesting dependence of the somatic mutational process on replication timing. On the other hand, the ratio of nonsynonymous to synonymous SNVs was higher than that for germ-line SNVs, suggesting weak purifying selection against deleterious mutations. Late-replicating regions contained many recurrently mutated genes without a signature of strong positive selection, supporting the notion that replication timing-dependent mutational process strongly influences the SNV spectrum of protein-coding genes. 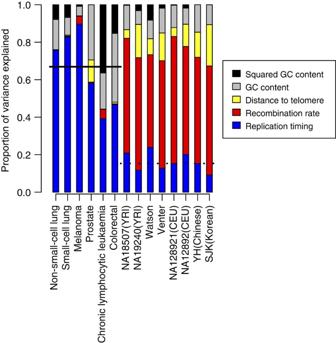Figure 1: Genomic features and SNV frequency. Bar plot showing the contribution of each genomic feature to the SNV frequency, determined by type III ANOVA. The SNV frequencies were square-root transformed. The contributions of the individual predictors to determining the SNV frequency are normalized to a sum of 1. The solid and dotted lines indicate the median contribution by replication timing to the somatic and the germ-line SNV data sets, respectively. The germ-line SNV data sets were from a compiled collection of various personal genome sequences (http://main.g2.bx.psu.edu; shared data library 'allSNP.txt'). The somatic SNV data sets are described inTable 1. Mutation frequency compared with replication timing We compiled 6 cancer SNV data sets containing 22 whole genome sequences from 6 cancer types: small-cell lung cancer, non-small-cell lung cancer, melanoma, prostate cancer, colorectal carcinoma, and chronic lymphocytic leukemia ( Table 1 ). The SNVs represent somatic events as they were identified from comparison of cancer and normal genomic sequences from the same patient. We also obtained germ-line SNVs from personal genome sequences. Among many mutation types, we focussed on SNVs because they are abundant and functionally important. We focussed on SNVs in non-CpG dinucleotide context because the cytosine in the CpG dinucleotide context is prone to mutation owing to a specific, methylation-dependent mechanism. Table 1 Cancer SNV data sets. Full size table We studied whether properties of a genomic region would influence the mutation rate. For 1Mb windows, we examined the following genomic features: genomic GC content, recombination rate, distance to the telomeres, and the replication timing during the S phase [22] , [23] , [24] . We focussed on functionally neutral or nearly neutral regions, in which the observed mutation frequencies would be influenced by the mutation rate only. We selected intergenic regions and removed from them potentially functional regions, such as transcription factor binding sites (TFBSs), open chromatin regions, and CpG islands. We removed regions with different replication timings in different cell types [24] . We conducted an ANOVA (type III) analysis to isolate contributions of individual genomic features to germ-line and cancer somatic SNVs while accounting for other features ( Fig. 1 ). For somatic SNVs, the replication timing explained over 60% of the total contributions. In contrast, for germ-line SNVs, replication timing explained <20% of the contributions, whereas recombination rate was a strong determinant of the SNV frequency, consistent with a previous study [25] . It seems that replication timing is a dominant determinant of the cancer somatic mutation rate, but it is a moderate determinant of the germ-line mutation rate. Figure 1: Genomic features and SNV frequency. Bar plot showing the contribution of each genomic feature to the SNV frequency, determined by type III ANOVA. The SNV frequencies were square-root transformed. The contributions of the individual predictors to determining the SNV frequency are normalized to a sum of 1. The solid and dotted lines indicate the median contribution by replication timing to the somatic and the germ-line SNV data sets, respectively. The germ-line SNV data sets were from a compiled collection of various personal genome sequences ( http://main.g2.bx.psu.edu ; shared data library 'allSNP.txt'). The somatic SNV data sets are described in Table 1 . Full size image We examined the rate by which the SNV frequency changes with replication timing. The neutral genomic regions were divided into ten groups, and a linear regression analysis was conducted to measure the rate of change ( Fig. 2 ; Supplementary Fig. S1 ). We found that the SNV frequency increased with replication timing significantly for both germ-line and somatic SNVs ( Fig. 2a–d ; Supplementary Fig. S1 ). We found that the SNV frequency increased with replication timing regardless of the substitution class ( Supplementary Fig. S2 ) or the CpG dinucleotide context ( Supplementary Fig. S3 ). However, the median of the regression coefficients, which reflect the rate of SNV frequency increase with replication timing progression, was 0.17 for somatic SNVs, drastically higher than 0.04 for germ-line SNVs ( Fig. 2e ). In other words, the somatic SNV frequency increased from the first (early replicating) to the tenth (late-replicating) group by 188%, whereas the germ-line SNV frequency increased only by 28% (See Methods for the calculating of the increase). For large-scale structural alterations involving genome copy-number changes, we did not observe drastic frequency changes with replication timing ( Supplementary Fig. S4 ). Together, these observations suggest that replication timing is a strong, general determinant of single-nucleotide mutation rate in cancer somatic cells. 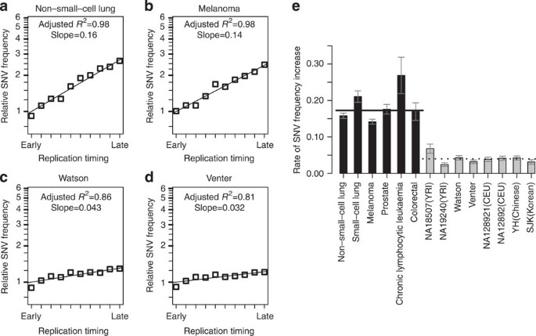Figure 2: SNV frequency compared with replication timing. (a–d) Scatter plot showing SNV frequencies (yaxis) among ten groups of genomic regions (xaxis), which were assigned the numbers fromx=0 (Early) tox=9 (Late) based on the replication timing. The adjusted R2and the regression coefficient (the slope) are shown. The slope of 0.16 for the melanoma genome (b) means that the SNV frequency increased from the first (x=0) to the tenth group (x=9) by (2(9−0)×0.16−1)×100%=171%. Theyaxis, in log2 scale, shows the relative SNV frequencies. (e) Bar plot showing the regression coefficients with the standard error (error bar). Solid and dotted lines represent the median regression coefficient for the somatic and germ-line SNV data sets, respectively. Figure 2: SNV frequency compared with replication timing. ( a – d ) Scatter plot showing SNV frequencies ( y axis) among ten groups of genomic regions ( x axis), which were assigned the numbers from x =0 (Early) to x =9 (Late) based on the replication timing. The adjusted R 2 and the regression coefficient (the slope) are shown. The slope of 0.16 for the melanoma genome ( b ) means that the SNV frequency increased from the first ( x= 0) to the tenth group ( x =9) by (2 (9−0)×0.16 −1)×100%=171%. The y axis, in log2 scale, shows the relative SNV frequencies. ( e ) Bar plot showing the regression coefficients with the standard error (error bar). Solid and dotted lines represent the median regression coefficient for the somatic and germ-line SNV data sets, respectively. Full size image We found strong associations between replication timing and SNV frequency in this study ( Fig. 2 ; Supplementary Fig. S1 ), in contrast to the recent conclusion of a weak association ( R 2 <0.5) [21] . Somatic SNVs are generally sparse in the cancer genome (<10 SNV Mb −1 ). The previous study [21] used 1 Mb windows for analysing SNV frequencies. We hypothesized that the low R 2 was in part due to high sampling variability. We did a linear regression analysis using SNV frequencies and replication timing, calculating R 2 using various interval sizes ranging from 10 kb to 10 Mb. We found that the R 2 increased with increasing interval sizes ( Supplementary Fig. S5 ), supporting the conclusion that small intervals together with sparse SNV occurrences would explain the low R 2 observed in the previous study. We note that the R 2 plateaued around ~0.5 at mega-base intervals; a simulation shows that R 2 should increase up to ~0.9 at these ranges ( Supplementary Fig. S5 ). This makes sense because homogeneity of genomic features would eventually break down when the intervals are increased linearly in the genome. When we combined 10 kb genomic intervals across the genome according to their replication timing, we detected R 2 values close to the simulated values ( Supplementary Fig. S5 ). It seems that combining intervals across the genomes, the strategy used in this study, would increase the effective interval size while minimizing genomic heterogeneity within the combined interval. SNV frequency in functional regions compared with replication timing We studied whether somatic SNV frequency would change with replication timing in functionally important regions, such as promoters, coding regions (coding), and introns. In these regions, SNV frequency tends to be lower than that in intergenic regions, confirming functional importance of these regions for biological processes, but within these functional regions, SNV frequency increased with replication timing ( Fig. 3a ; Supplementary Fig. S6 ). Thus, the influence of replication timing on the mutational rate was clear in functional regions. 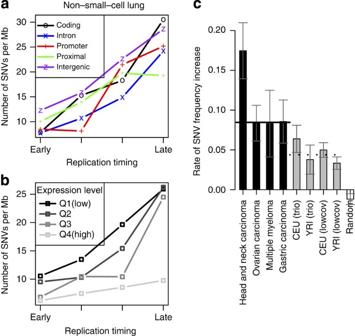Figure 3: SNV frequency compared with replication timing for functional regions. (a) Scatter plot showing SNV frequencies (yaxis) as a function of replication timing (xaxis) in the four types of functional regions (lines): intronic (intron), coding sequences (coding), 0–1,000 bp upstream of TSS (promoter), 1,000–5,000 bp upstream of TSS (proximal), and >5000 upstream of TSS (intergenic). Putative functional sites were not removed from the intergenic regions. The SNV data set is from the non-small-cell lung cancer sample (Table 1). (b) Somatic SNV frequencies (yaxis) in intronic regions as a function of replication timing (xaxis) and gene expression level (lines). We removed regions within 50 bp of the exon–intron junction or regions with significant DNase I hypersensitivity. We used gene expression data generated using Affymetrix GeneChip microarrays4. (c) Bar plot showing the regression coefficients with the standard error (error bar) for synonymous cancer and germ-line SNVs. A linear regression analysis was conducted using the log2 SNV frequency and the replication timing as the response and the predictor variable, respectively. The solid and dotted lines indicate the median regression coefficient for somatic and germ-line SNV data sets, respectively. The somatic SNV data sets are described inTable 1. The germ-line SNV data were from high-coverage trios (trio) and low-coverage population (lowcov) sequencing data from the pilot phase of the 1,000 genome project38. CEU (U.S. Utah residents with ancestry from northern and western Europe); YRI (The Yoruba in Ibadan, Nigeria). We included ~170,000 randomly generated synonymous SNVs (random). Figure 3: SNV frequency compared with replication timing for functional regions. ( a ) Scatter plot showing SNV frequencies ( y axis) as a function of replication timing ( x axis) in the four types of functional regions (lines): intronic (intron), coding sequences (coding), 0–1,000 bp upstream of TSS (promoter), 1,000–5,000 bp upstream of TSS (proximal), and >5000 upstream of TSS (intergenic). Putative functional sites were not removed from the intergenic regions. The SNV data set is from the non-small-cell lung cancer sample ( Table 1 ). ( b ) Somatic SNV frequencies ( y axis) in intronic regions as a function of replication timing ( x axis) and gene expression level (lines). We removed regions within 50 bp of the exon–intron junction or regions with significant DNase I hypersensitivity. We used gene expression data generated using Affymetrix GeneChip microarrays [4] . ( c ) Bar plot showing the regression coefficients with the standard error (error bar) for synonymous cancer and germ-line SNVs. A linear regression analysis was conducted using the log2 SNV frequency and the replication timing as the response and the predictor variable, respectively. The solid and dotted lines indicate the median regression coefficient for somatic and germ-line SNV data sets, respectively. The somatic SNV data sets are described in Table 1 . The germ-line SNV data were from high-coverage trios (trio) and low-coverage population (lowcov) sequencing data from the pilot phase of the 1,000 genome project [38] . CEU (U.S. Utah residents with ancestry from northern and western Europe); YRI (The Yoruba in Ibadan, Nigeria). We included ~170,000 randomly generated synonymous SNVs (random). Full size image We wondered whether the association between SNV frequency in genic regions and replication timing was a spurious correlation driven by transcription level, as transcription-coupled repairs are known to influence somatic SNV frequencies in cancer cells [3] , [4] . Consistent with these previous observations, SNV frequency in functionally neutral intronic regions decreased with increasing transcription level. However, even after accounting for transcription level, SNV frequency still increased with replication timing ( Fig. 3b ). This is consistent with previous findings [26] and rules out the possibility that the observed association between SNV frequency and replication timing was caused by transcription level. Replication timing influences the mutation rate in both genic and inter-genic regions and is a more general determinant of mutation rate than transcription-coupled repair, whose influence on the mutation rate is limited to genic regions. We further examined the relationship between the mutational processes in the protein-coding regions and replication timing. We focussed on synonymous SNVs, to minimize influence of selection. Synonymous SNVs can be functionally important and evolutionarily constrained [27] , [28] , so we removed from the analysis coding regions whose synonymous substitutions are evolutionarily constrained among mammals and regions that overlap with DNase I hypersensitive sites. As synonymous SNVs are sparse in individual cancer genomes, we obtained cancer exome data sets from large cohorts of ovarian carcinoma, head and neck carcinoma, gastric carcinoma, and multiple myeloma and pooled the mutation data across patients for each cohort ( Table 1 ). The synonymous SNV frequency increased with replication timing, with a higher rate for somatic SNVs than for germ-line SNVs ( Fig. 3c ; Supplementary Fig. S7 ). These results underscore strong influences of replication timing on mutations in protein-coding regions. Global selection landscape of somatic SNVs We characterized the selection pressure on somatic mutations in cancer cells. We compared the abundance of functional mutations with that of neutral mutations, reasoning that most functional mutations would be deleterious and would be depleted in the presence of selection pressure against deleterious mutations. We focussed on the protein-coding regions, where functional consequences of the mutations can be reasonably assessed from the resulting amino-acid sequences, that is, synonymous or nonsynonymous. We calculated the ratio between synonymous and nonsynonymous SNVs for four cancer somatic SNV data sets and for four germ-line SNV data sets. For germ-line SNVs, nonsynonymous SNVs are significantly depleted compared with the expected by chance, suggesting strong purifying selection against protein-coding mutations ( Fig. 4a ). For cancer somatic SNVs, the ratios between nonsynonymous and synonymous SNVs were close to the expected by chance, suggesting that the selection pressure against somatic nonsynonymous SNVs in cancer cells is much weaker than that in germ cells. Many nonsynonymous SNVs, especially missense SNVs, have small effects on the protein structure and functionally inconsequential [29] . We repeated the analysis with a subset of nonsynonymous SNVs with strong functional consequences: nonsense SNVs that truncate more than half of the gene product by premature stop codons. We found the same trend that these nonsense SNVs were significantly depleted only for germ-line SNVs, but not for somatic SNVs ( Fig. 4b ). It seems that selection pressure against deleterious protein-coding mutations is weak in cancer somatic cells. Possible explanations are provided in Discussion. 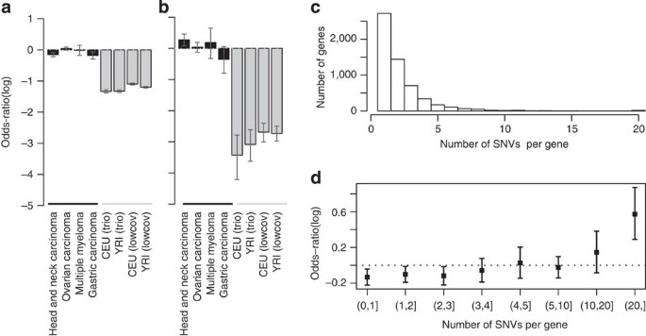Figure 4: Selection signature for protein-coding SNVs. (a) For each of the four germ-line and the four somatic SNV data sets, the ratio of nonsynonymous to synonymous SNVs was calculated, and was compared against the ratio from random SNVs in coding regions. We calculated log odds-ratios (yaxis), where positive and negative values would mean enrichment and depletion of nonsynonymous SNVs, respectively. The error bars indicate the 95% CI. In (b), we focussed on nonsense mutations that truncate more than half of the gene product by introducing premature stop codons. (c) Histogram showing the distribution of genes with varying number of SNVs. Genes with at least one synonymous or nonsynonymous SNV are shown. Thexaxis was truncated at 20. (d) The log odds-ratios (yaxis) as a function of the number of SNVs per gene (xaxis). Figure 4: Selection signature for protein-coding SNVs. ( a ) For each of the four germ-line and the four somatic SNV data sets, the ratio of nonsynonymous to synonymous SNVs was calculated, and was compared against the ratio from random SNVs in coding regions. We calculated log odds-ratios ( y axis), where positive and negative values would mean enrichment and depletion of nonsynonymous SNVs, respectively. The error bars indicate the 95% CI. In ( b ), we focussed on nonsense mutations that truncate more than half of the gene product by introducing premature stop codons. ( c ) Histogram showing the distribution of genes with varying number of SNVs. Genes with at least one synonymous or nonsynonymous SNV are shown. The x axis was truncated at 20. ( d ) The log odds-ratios ( y axis) as a function of the number of SNVs per gene ( x axis). Full size image Recurrence of mutations and mutational heterogeneity We examined the distribution of SNVs across 10,222 protein-coding, non-overlapping genes ( Fig. 4c ). Of these, 5,673 genes incurred at least one SNV in the protein-coding region. We compared the observed recurrence to the expected when mutations were randomly assigned to each gene according to the protein-coding region size. The number of genes with 1–2 (sporadic) SNVs was 4,164, significantly lower than expected (95% range=4,389–4,568). However, the number of genes incurring >10 (recurrent) SNVs was 50, significantly higher than expected (95% range=19–33). It seems that the same gene tends to be mutated recurrently. We examined the selection pressure as an explanation for the increased SNV recurrence. Among the 4,164 genes with sporadic mutations, there was a slight depletion of nonsynonymous SNVs compared with synonymous SNVs, suggesting weak negative selection. Among the 50 genes with recurrent SNVs, nonsynonymous SNVs were in excess of synonymous SNVs, suggestive of positive selection ( Fig. 4d ). When we examined the selection pressure for each gene, six genes showed evidence for strong positive selection, that is, showing great excess of nonsynonymous SNVs (the ratio >20) ( Fig. 5a ). Four of them were well-known cancer drivers, TP53, BRCA1, BRCA2 and NRAS. The other two genes, UTRN and RYR1, were not registered in the cancer gene consensus database but were implicated in cancer pathways [30] . Also, UTRN is known to be mutated in multiple cancers [31] . 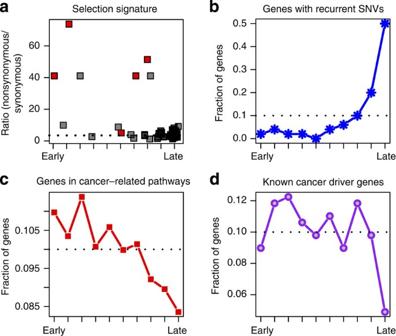Figure 5: Replication timing and cancer driver genes. Genes were divided into ten equal-sized groups (xaxis) according to the replication timing. Replication timing was averaged over each gene. (a) The ratio of nonsynonymous to synonymous SNVs for individual genes that incur recurrent (>10) SNVs. To stabilize the estimate, we added the genome-wide average of the nonsynonymous and synonymous SNVs per gene to the numerator and the denominator of the ratio. The red-coloured points denote known cancer driver genes from the cancer gene consensus database. (b) The fraction of genes with recurrent SNVs. (c) The fraction of genes involved in cancer pathways. (d) The fraction of known cancer driver genes. Dotted lines aty=0.1 indicate the fraction of genes evenly distributed across replication timing. Figure 5: Replication timing and cancer driver genes. Genes were divided into ten equal-sized groups ( x axis) according to the replication timing. Replication timing was averaged over each gene. ( a ) The ratio of nonsynonymous to synonymous SNVs for individual genes that incur recurrent (>10) SNVs. To stabilize the estimate, we added the genome-wide average of the nonsynonymous and synonymous SNVs per gene to the numerator and the denominator of the ratio. The red-coloured points denote known cancer driver genes from the cancer gene consensus database. ( b ) The fraction of genes with recurrent SNVs. ( c ) The fraction of genes involved in cancer pathways. ( d ) The fraction of known cancer driver genes. Dotted lines at y= 0.1 indicate the fraction of genes evenly distributed across replication timing. Full size image It is important to note that these 6 genes make up only 12% of the recurrently mutated genes, failing to account for the other 88%. We studied whether replication timing-dependent mutational heterogeneity contributed to these recurrent mutations. With replication timing progression, the fraction of the recurrently mutated (>10 SNVs) genes increased ( Fig. 5b ), but the fraction of genes with signatures of positive selection actually decreased ( Fig. 5a ). Furthermore, late-replicating regions were depleted of genes implicated in cancer pathways, that is, whose mutations would likely impact tumorigenesis ( Fig. 5c ) or known cancer driver genes ( Fig. 5d ). In other words, genes in late-replicating regions can be recurrently mutated without influences of selection, underscoring the importance of replication timing-dependent genome organization in shaping the mutation spectrum of cancer genomes. In summary, we found important differences between the evolutionary dynamics of cancer somatic cells and that of the whole organisms. In cancer cells, the dependence of the mutation rate on replication timing is stronger, but selection against coding mutations is weaker than in germ-line cells. Many genes in late-replicating regions were recurrently mutated without signatures of positive selection. We conclude that the mutation spectrum of the cancer genome can be influenced by a replication timing-dependent mutational process. Recent studies have shown the importance of genome organization in shaping the landscape of large-scale structural alterations [17] , [18] . Because large-scale alterations are likely to hit functional regions, it is difficult to separate the influence of the mutation from that of the selection. For example, a previous study [18] showed that deletions would increase, but amplifications would decrease with replication timing. Such trends can be explained by the distribution of functionally different genes across the replication timing [32] . Early replicating regions contain growth- and development-related genes, whose amplifications can cause cellular proliferations. Late-replicating regions contain many tissue-specific genes; deletion of these genes are more likely to be tolerated than deletion of genes in early replicating regions. For SNVs, it is straightforward to distinguish functional from neutral ones and that the relationship between genome organizations and the mutational processes can be directly tested, largely independent of selection. We found significantly lower selection pressure against coding mutations in cancer somatic cells than in germ cells. This makes an intuitive sense because beneficial mutations at the level of multicellular organisms would be rarer than those at the level of their individual cells, consistent with the idea of the cost of complexity [33] . Furthermore, somatic mutations would be restricted to the progeny of the mutated cells, but germ-line mutations would be propagated to all cells in an organism, increasing the chance of exerting deleterious effects in some cell types. The observation that the somatic mutation rate per generation is higher than the germ-line mutation rate [16] raises an interesting notion that multicellular organisms have evolved to optimize somatic and germ-line mutation rates, so that an organism can keep individual cells viable during its lifetime while passing sufficiently intact genetic information to its offspring. What is the mechanistic basis for strong dependence of the SNV frequency on replication timing in cancer somatic cells but not in germ cells? First, there are likely to be additional layers of repair mechanisms in germ cells, which would buffer replication timing-dependent accumulation of mutations. Supporting this, germ-line mutation rates are known to be lower than somatic mutation rates [16] . The exact mechanism would become clear with advances in our understanding of the DNA repair in germ and somatic cells. Second, high genome instability and external DNA damaging assaults, such as tobacco and ultraviolet radiation exposures, can cause many somatic mutations in cancer cells. This would likely overwhelm the capacity of DNA damage recognition and repair processes and only a subset of mutations will be repaired. Early-replicating regions tend to have open chromatin structure, so they are more likely to be accessible to repair factors than late-replicating regions [23] . We speculate that preferential repair of early replicating regions will be heightened when the system is overwhelmed, resulting in greater heterogeneity in mutation frequency between early and late-replicating regions. Why are cancer-related genes depleted in late-replicating regions? Because cancers usually occur beyond the reproductive age, cancer traits would not be under direct selection pressure. However, many cancer-related genes are often involved in fundamental cellular processes such as development, cell cycle, and DNA repair, and these genes tend to be in early replicating regions [34] . A recent study has shown that replication timing is an evolvable property [35] . We speculate that, during evolution, it was advantageous to expedite the replication timing of these genes to decrease their mutation rate, thus maintaining factors necessary for fundamental cellular processes. On other hand, late-replicating regions tend to contain tissue-specific or lowly expressed genes, likely because their mutations would be more likely to be tolerated than development-related, cancer-causing genes. Replication timing is highly plastic and often changes, depending on the cell type [24] . Replication timing data with matching cell types are not available for most of the cancer genomes examined in this study. We therefore employed an alternative strategy: to focus on genomic regions that maintain constant replication timing across cell types. This strategy was utilized in a recent study that successfully uncovered the relationship between large-scale structural alterations and replication timing [18] . We found that regions that maintain consistent replication timing across the three nonmalignant cell lines (BG02, BJ, and GM06990) tended to maintain the same replication timing in the cancer cell line (K562), suggesting that these regions would also likely maintain the same replication timing in the cancer samples analysed in this study ( Supplementary Fig. S8 ). Importantly, variations in the replication timing would likely obscure rather than exaggerate the true correlation between SNV frequency and replication timing; supporting this, the correlation was weaker when the analysis included regions with variable replication timing across cell types ( Supplementary Fig. S9 ). We speculate that the correlation would be stronger with matching replication timing data. The current study can be expanded in several ways. First, this study examined SNV spectrums in ten different tumour types, many of which were carcinomas which tend to be caused by heavy exposure to DNA damaging agents, such as tobacco and ultraviolet exposure. Indeed, the rate of the replication timing-dependent SNV frequency increase varied ( Fig. 2 ), suggesting that not all cancers are equally influenced by replication timing-dependent mutational process. Furthermore, there are hundreds of cancer types. The current effort to sequence thousands of samples in 50 tumour types would ascertain whether the observations of this study are general for all cancer types [11] . Second, we would like to conduct a systematic dissection of how mutational heterogeneity is influenced by multiple factors, such as the tissue type, exposure to mutagens, age of the host, and so on [36] . Particularly, do differences in the mutational process lead to different evolutionary paths and different clinical outcomes? Third, we would like to characterize the selection pressure for individual genes. For this study as well as previous studies [4] , [37] , we pooled SNVs across genes to infer strength of selection because of sparseness of somatic SNVs (<10 SNVs Mb −1 ); such pooling will become less necessary with sufficiently large numbers of sequenced cancer genomes. Many of these fundamental questions in cancer genetics can be elucidated in part by the current effort to map the mutations in thousands of cancer samples [11] . Genome data sets We obtained data sets of 22 cancer genomes representing 6 different cancer types ( Table 1 ). They were generated by six independent studies using three sequencing platforms, so it is unlikely that study-specific, platform-specific biases influenced the conclusion of this study. Twenty-one of the 22 cancer genomes were sequenced with >25×coverage, estimated to be sufficient for high accuracy and precision of SNV detection [2] . We obtained 450 exomes representing four different cancer types for analyses of protein-coding mutations ( Table 1 ). We used germ-line SNVs from personal genome sequences ( http://main.g2.bx.psu.edu ; shared data library 'allSNP.txt') and from the pilot 1000 genome project [38] ( http://www.1000genomes.org ). Germ-line SNVs were used if the human reference genome allele were the same as the ancestral allele provided by the data sets. We also generated ~170,000 and ~610,000 synonymous and nonsynonymous SNVs from random nucleotide substitutions in the coding regions. We removed mutations in the CpG dinucleotide context from the analysis, except when examining mutations of specific substitution classes and those of CpG dinucleotide context. Replication timing We obtained genome-wide maps of replication timing [24] , which were generated by sequencing genomic DNAs replicated during six cell-cycle stages (G1, S1, S2, S3, S4 and G2) for four Encyclopedia of DNA Elements (ENCODE) cell lines: embryonic stem cell (BG02), fibroblast (BJ), lymphoblastoid cells (GM06990), and myelogenous leukaemic cells (K562). We used a wavelet-smoothed, weighted average signal whose high and low values indicate early and late replication during the S phase, respectively ( http://genome.ucsc.edu/ENCODE , 'Repli-seq track') and divided the genome into ten equal-sized groups: [25.9] [25.9,33.8] [33.8,40.0] [40.0,45.6] [45.6,50.7] [50.7,55.5] [55.5,60.3] [60.3,65.4] [65.4,70.9] [70.9] or, in some cases, four groups: [37.0], [37.0, 50.7], [50.7, 62.9], and [62.9]. We focussed on genomic regions that maintain similar replication timing between cell types for this analysis as follows. First, for each 1 kb genomic window, we calculated the stage where 50% of the genomic region was replicated. We combined the S1 stage with the G1 stage, and the S4 stage with the G2 stage, as previously done [24] . The correspondence between these four stages, S1, S2, S3 and S4 and the 10 groups, which were used for most of the analyses, are shown in Supplementary Fig. S10 . A genomic region was considered to be cell-type invariant if its stages across the 4 ENCODE cell lines were the same or different by one stage, that is, S1–S2, S2–S3 or S3–S4. Genomic features All genomic coordinates were based on the human genome build of hg18; the hg19 coordinates were remapped to the hg18 coordinates using the UCSC liftOver program ( http://genome.ucsc.edu ). DNase I hypersensitive sites and transcription factor binding sites, indicative of functional regulatory regions, were obtained from ENCODE ( http://genome.ucsc.edu/ENCODE/ ). We obtained recombination rates from International HapMap Project: ( http://hapmap.ncbi.nlm.nih.gov/ ) and averaged them over non-overlapping 100 kb windows across the genome. We focussed on autosomes only. Definitions of individual genes were based on the NCBI gene definition (build 36). We focussed on genes that have an unambiguous annotation of a coding sequence from the consensus coding sequence project (CCDS) [39] . We removed genes that overlapped with other genes or those whose tested coding sequences were <100 bp in size. Cancer driver genes were obtained from the cancer gene consensus database ( http://www.sanger.ac.uk/genetics/CGP/Census /) (March 2010). Genes implicated in cancer pathways based on gene expression modules were obtained from Broad Institute Gene Sets [30] ( http://www.broadinstitute.org/gsea/ ) ('c4.cm.v3.0.entrez.gmt'). Partitioning genomes into functional or neutral regions We identified functionally neutral, intergenic regions as follows. First, from the whole genome, we removed all genic regions and regions that are 5,000 bp upstream of the transcription start site (TSS). The canonical gene start site was used as an approximate estimate of the TSS. We selected regions defined as intergenic by all of the three gene annotation sources: Gencode [40] Genes ( http://www.gencodegenes.org ), Refseq Genes ( http://genome.ucsc.edu ), and UCSC Genes ( http://genome.ucsc.edu ). Second, we removed CpG islands, which may not evolve neutrally, and difficult-to-map regions identified by the ENCODE project, which tend to contain highly repetitive sequences. Third, we removed putative regulatory regions marked by DNase I hypersensitive regions and transcription factor binding sites and their 100 bp flanking regions. The functional regions examined in this study were introns, coding sequences (coding), promoters (0–1,000 bp from TSS), and proximal (1,000–5,000 bp from TSS). We focussed on regions classified concordantly by all of the three gene definitions. Coding regions (coding) were obtained from the consensus CDS project [39] . Analysis All analyses were performed in R ( http://www.r-projects.org ). Genomic interval analyses were performed using R/intervals. G/C and CpG sites were identified using R/BSgenome and R/Biostrings ( http://www.bioconductor.org ). We conducted ANOVA type III tests using the drop1 function in R. Each interval was weighted according to its genomic size. We conducted a simple linear regression analysis using the lm function in R. We used the log2-transformed SNV frequencies as the dependent variable and the numbers from x =0 to x =9, corresponding to the 10 genomic region groups, as the predictor variable. Because of the logarithmic transformation, the regression coefficient, or the slope, would indicate the rate of proportional rather than absolute changes in SNV frequency with replication timing progression [41] . For example, a slope of 0.1 would mean that the SNV frequency increased from the first ( x= 0) to the tenth group ( x =9) by (2 (9−0)×0.1 −1)×100%=86%. The SIFT module as implemented in the Galaxy platform ( http://main.g2.bx.psu.edu ) [42] was used to classify protein-coding SNVs as synonymous or nonsynonymous [29] . Odds-ratio and its confidence intervals were computed using the Fisher's test function in R. How to cite this article: Woo Y.H. and Li W.-H. DNA replication timing and selection shape the landscape of nucleotide variation in cancer genomes. Nat. Commun. 3:1004 doi: 10.1038/ncomms1982 (2012).